A common East-AsianALDH2mutation causes metabolic disorders and the therapeutic effect of ALDH2 activators Obesity and type 2 diabetes have reached pandemic proportion. ALDH2 (acetaldehyde dehydrogenase 2, mitochondrial) is the key metabolizing enzyme of acetaldehyde and other toxic aldehydes, such as 4-hydroxynonenal. A missense Glu504Lys mutation of the ALDH2 gene is prevalent in 560 million East Asians, resulting in reduced ALDH2 enzymatic activity. We find that male Aldh2 knock-in mice mimicking human Glu504Lys mutation were prone to develop diet-induced obesity, glucose intolerance, insulin resistance, and fatty liver due to reduced adaptive thermogenesis and energy expenditure. We find reduced activity of ALDH2 of the brown adipose tissue from the male Aldh2 homozygous knock-in mice. Proteomic analyses of the brown adipose tissue from the male Aldh2 knock-in mice identifies increased 4-hydroxynonenal-adducted proteins involved in mitochondrial fatty acid oxidation and electron transport chain, leading to markedly decreased fatty acid oxidation rate and mitochondrial respiration of brown adipose tissue, which is essential for adaptive thermogenesis and energy expenditure. AD-9308 is a water-soluble, potent, and highly selective ALDH2 activator. AD-9308 treatment ameliorates diet-induced obesity and fatty liver, and improves glucose homeostasis in both male Aldh2 wild-type and knock-in mice. Our data highlight the therapeutic potential of reducing toxic aldehyde levels by activating ALDH2 for metabolic diseases. Obesity and type 2 diabetes have reached pandemic levels. The 2019 International Diabetes Federation reported that there were 463 million people living with diabetes worldwide. This number is projected to increase rapidly to 578 million in 2030 [1] . East Asia and South Asia, the most populous regions in the world, are expected to be the major contributors of new cases [1] . This pandemic is primarily caused by a high-calorie diet enriched in fat and sugar, sedentary lifestyle, and their interaction with genetic factors [1] , [2] . Approximately 36% of East Asians (560 million) or nearly 8% of the global population, carry an inactivating Glu504Lys missense mutation of the ALDH2 gene [3] . This mutation results in a reduction of the ALDH2 enzymatic activity by 60–80% in heterozygous carriers and ~90% in homozygous carriers [4] . People carrying this mutation exhibit sensitivity to alcohol, with presentations ranging from facial flushing, headache, and tachycardia due to a rapid increase in circulating acetaldehyde concentrations [5] , [6] . Epidemiological studies suggest a correlation between this inactivating mutation and several diseases including oral cancer, esophageal cancers, and blood and solid tumors associated with Fanconi anemia [7] , [8] . Importantly, several large-scale meta-analyses of genome-wide association studies revealed that this inactivating mutation is strongly associated with type 2 diabetes [9] , body mass index [10] , and serum lipids [11] in East Asians. A validation study further confirmed a close association of the ALDH2 mutant variant with visceral fat distribution in 2958 Chinese subjects [12] . In addition, carriers of the inactivating ALDH2 variant had 2-3 times increased risk of non-alcoholic fatty liver disease among Japanese subjects [13] . The ALDH2 gene encodes mitochondrial aldehyde dehydrogenase 2 (ALDH2), a major acetaldehyde-metabolizing enzyme responsible for ~95% acetaldehyde metabolism due to its low Km for acetaldehyde [14] . Acetaldehyde is produced by alcohol dehydrogenase (ADH) following alcohol ingestion. Acetaldehyde can also be generated endogenously from the intermediate metabolisms or by gut microbial flora [15] . Air pollution, thermal degradation of plastics, and spoiled food are also sources of toxic aldehyde [16] , [17] , [18] . Acetaldehyde is listed as group I carcinogen by the International Agency for Research on Cancer [19] . In addition to acetaldehyde, ALDH2 also metabolizes various bioactive toxic aldehydes, including acrolein, malondialdehyde and 4-hydroxynonenal (4-HNE). Among these bioactive aldehydes, the most intensively studied one has been 4-HNE, a lipid peroxidation product that forms covalent adduct to macromolecules such as protein, lipid and DNA, causing cellular damage [20] , [21] , [22] , [23] , [24] . With the advent of high-throughput screening, a small molecule, Alda-1 , was identified as an activator for both the wild-type ALDH2 and mutant ALDH2 enzymes [25] . Based on X-ray crystallography and enzyme kinetics, the binding of Alda-1 partially blocks the exit tunnel of substrates, thus increasing the likelihood of productive encounters between reaction intermediate and the catalytic site [26] . Administration of Alda-1 has been effective to treat myocardial infarction, aortic aneurysm, atrial fibrillation, Alzheimer’s disease and nociceptive pain by enhancing the clearance of 4-HNE in rodents [27] , [28] , [29] , [30] . The discovery of ALDH2 activators offers an opportunity to test the therapeutic potential of reducing toxic aldehydes for treating a variety of diseases. AD-9308 is a highly water soluble and orally bioavailable prodrug of a potent and highly selective ALDH2 activator, AD-5591 , a new generation ALDH2 activator that has the improved biological activities and pharmacological properties compared to Alda-1 [31] . In this study, we used Aldh2 homozygous knock-in (KI) and heterozygous knock-in (HE) mice, which mimic the East Asian-specific Glu504Lys mutation, to evaluate the effect of this mutation on diet-induced obesity, glucose homeostasis, fatty liver, and serum lipids, and tested the therapeutic effect of a feasible ALDH2 activator AD-5591 by dosing its prodrug AD-9308 for treating metabolic disorders. Aldh2 KI mice carrying the East Asian-specific Glu504Lys mutation were prone to develop diet-induced obesity and fatty liver To assess the effect of the East Asian-specific ALDH2 Glu504Lys mutation on diet-induced obesity and related metabolic traits, Aldh2 KI, HE, and WT mice were placed on high-fat high-sucrose diet (HFHSD) for 24 weeks since the age of 4 weeks. At the end of study, the body weights of Aldh2 KI, HE and WT mice were 41.66 ± 1.40, 41.65 ± 1.13, and 36.95 ± 0.96 g respectively (Fig. 1a , P -for-trend = 0.0096). However, no difference of body weight gain was observed between Aldh2 KI and WT mice fed a chow diet. Aldh2 KI, HE, and WT mice fed on HFHSD also had more white fat, including perigonadal fat (2.76 ± 0.27 vs. 2.41 ± 0.16 vs. 1.63 ± 0.13 g, P -for-trend < 0.001), inguinal fat (1.69 ± 0.16 vs. 1.55 ± 0.12 vs. 1.24 ± 0.11 g, P -for-trend = 0.011), mesenteric fat (0.85 ± 0.09 vs. 0.87 ± 0.05 vs. 0.32 ± 0.05 g, P -for-trend = 0.018), and a trend of increased liver weight (1.84 ± 0.07 vs. 1.70 ± 0.13 g vs. 1.61 ± 0.07 g, P -for-trend = 0.069), but less brown adipose tissue (BAT) weight (0.12 ± 0.009 vs. 0.17 ± 0.0.02 vs. 0.17 ± 0.01 g, P -for-trend = 0.006) ( Fig. 1b ) at the age of 24 weeks. No such differences were found between Aldh2 KI and WT mice on chow diet. Body composition analysis revealed significantly increased fat mass of Aldh2 KI and HE compared with the WT mice fed on HFHSD (12.40 ± 1.00, 10.04 ± 1.09, 8.41 ± 0.78 g, P -for-trend = 0.0058) (Fig. 1c ) at the age of 24 weeks. There was no difference of fat mass between Aldh2 KI and WT mice on a chow diet. 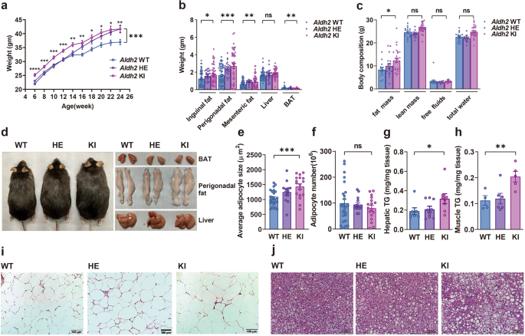Fig. 1:Aldh2(acetaldehyde dehydrogenase 2) knock-in (KI) mice mimicking human Glu504Lys mutation were prone to develop diet-induced obesity, glucose intolerance, insulin resistance, and fatty liver. Body weight ofAldh2, homozygous knock-in (KI) and heterozygous KI (HE), and wild-type (WT) mice onahigh-fat high sucrose diet (HFHSD) (n= 24:36: 21; repeated measure analysis of variance [ANOVA]P= 0.0002) andbweights of inguinal, perigonadal, and mesenteric fat, the liver, and brown adipose tissue (BAT) of theAldh2WT and KI mice (n= 63:24:48;P-for-trend = 0.011, <0.001, 0.0065, 0.053, and 0.0069 respectively).cBody composition ofAldh2WT and KI mice (n= 16:17:22 in triplicates;P-for-trend = 0.02, 0.09, 0.77, 0.10 and respectively).dGross appearance if mice, BAT, perigonadal fat and liver.eAverage adipocyte size (P-for-trend = 0.0003) andfadipocyte number in the perigonadal fat pad of theAldh2homozygous KI, HE, and WT mice (n= 24:14:17;P-for-trend = 0.030).gHepatic triglyceride content of theAldh2homozygous KI, HE, and WT mice (n= 7:9:8 in duplicates;P-for-trend = 0.034).hMuscle triglyceride content in theAldh2homozygous KI and HE, and WT mice on HFHSD (n= 7:8:8;P-for-trend = 0.0086).iRepresentative H&E (hematoxylin and eosin) stain of the perigonadal fat inAldh2KI, HE, and WT mice.jRepresentative H&E staining of livers from theAldh2homozygous KI and HE, and WT mice. The scale bar of is 100 µm. The scale bar of is 100 µm. Figures (a–c,e–h) were analyzed tests for linear trends. Figure (a) was further analyzed using repeated measures ANOVA. All data are presented as mean and standard error (S.E.M.). Thenvalues represent biological repeats and the number of technical repeats were expressed as duplicates or triplicates. The asterisks indicate two-sided *P< 0.05, **P< 0.01, ***P< 0.001. Figure 1d showed the representative gross appearance of mice, BAT, perigonadal fat, and liver at the age of 24 weeks. There was dose-dependent increase in adipocyte size (1039.2 ± 54.6, 1247.9 ± 91, 1433.6 ± 91.22 μm 2 , P -for-trend = 0.0013) among three genotype although there was no difference in the number of adipocytes (Fig. 1 e, f), indicating hypertrophy rather than hyperplasia of white adipose tissue. Aldh2 KI and HE mice also had significantly higher hepatic triglycerides contents and more severe hepatic steatosis than the WT mice on HFHSD (0.32 ± 0.05 vs, 0.21 ± 0.03 vs. 0.19 ± 0.03 mg/mg liver tissue, P -for-trend = 0.034) (Fig. 1g, j ) at the age of 24 weeks. The skeletal muscle triglycerides content is also higher in Aldh2 KI and HE mice compared to WT mice (0.18 ± 0.01 vs, 0.15 ± 0.02 vs. 0.10 ± 0.01 mg/mg muscle tissue, P -for-trend = 0.0051) (Fig. 1h ). Hematoxylin and eosin (H&E) stain of perigonadal fat showed hypertrophic adipocytes with more crown-like necrosis in Aldh2 KI and HE mice compared with controls at the age of 24 weeks (Fig. 1i ). These results suggest that the East Asian-specific ALDH2Glu504Lys mutation promoted HFHSD-induced obesity and fatty liver in mice. Fig. 1: Aldh2 (acetaldehyde dehydrogenase 2) knock-in (KI) mice mimicking human Glu504Lys mutation were prone to develop diet-induced obesity, glucose intolerance, insulin resistance, and fatty liver. Body weight of Aldh2 , homozygous knock-in (KI) and heterozygous KI (HE), and wild-type (WT) mice on a high-fat high sucrose diet (HFHSD) ( n = 24:36: 21; repeated measure analysis of variance [ANOVA] P = 0.0002) and b weights of inguinal, perigonadal, and mesenteric fat, the liver, and brown adipose tissue (BAT) of the Aldh2 WT and KI mice ( n = 63:24:48; P -for-trend = 0.011, <0.001, 0.0065, 0.053, and 0.0069 respectively). c Body composition of Aldh2 WT and KI mice ( n = 16:17:22 in triplicates; P -for-trend = 0.02, 0.09, 0.77, 0.10 and respectively). d Gross appearance if mice, BAT, perigonadal fat and liver. e Average adipocyte size ( P -for-trend = 0.0003) and f adipocyte number in the perigonadal fat pad of the Aldh2 homozygous KI, HE, and WT mice ( n = 24:14:17; P -for-trend = 0.030). g Hepatic triglyceride content of the Aldh2 homozygous KI, HE, and WT mice ( n = 7:9:8 in duplicates; P -for-trend = 0.034). h Muscle triglyceride content in the Aldh2 homozygous KI and HE, and WT mice on HFHSD ( n = 7:8:8; P -for-trend = 0.0086). i Representative H&E (hematoxylin and eosin) stain of the perigonadal fat in Aldh2 KI, HE, and WT mice. j Representative H&E staining of livers from the Aldh2 homozygous KI and HE, and WT mice. The scale bar of is 100 µm. The scale bar of is 100 µm. Figures ( a – c , e – h ) were analyzed tests for linear trends. Figure ( a ) was further analyzed using repeated measures ANOVA. All data are presented as mean and standard error (S.E.M.). The n values represent biological repeats and the number of technical repeats were expressed as duplicates or triplicates. The asterisks indicate two-sided * P < 0.05, ** P < 0.01, *** P < 0.001. Full size image Aldh2 KI mice had reduced energy expenditure and impaired adaptive thermogenesis Energy expenditure measured by indirect calorimetry showed that Aldh2 KI and HE mice had significantly lower energy expenditure, especially in active (dark) phase at the age of 8–10 weeks (Fig. 2a ) than WT mice. In addition, indirect calorimetry also revealed Aldh2 KI and HE mice have higher respiratory exchange rate (RER) compared with WT mice (Supplementary Fig. 1 ), suggesting reduced fatty acid utilization. There was no difference in accumulative food intake over three weeks among three genotypes (Fig. 2b ). These data indicated Aldh2 KI and HE mice were prone to diet-induced obesity due to reduced energy expenditure but not intake. Fig. 2: Aldh2 (acetaldehyde dehydrogenase 2) knock-in mice mimicking human Glu504Lys mutation have reduced energy expenditure and adaptive thermogenesis. a Energy expenditure ( n = 19:27:13; repeated measures analysis of variance [ANOVA] P < 0.0001), b accumulative food intake for three weeks ( n = 8:24:10; repeated measures ANOVA P = 0.70), c wheel rotations ( n = 9:13:5; P -for-trend = 0.55), d distance traveled ( n = 5:20:7 P -for-trend = 0.27), and e behaviors monitored by HomeCage systems ( n = 5:20:7; P -for-trend = 0.88, 0.54, 0.48, 0.12, 0.31, 0.92, 0.65, 0.19, and 0.52 respectively) of the Aldh2 homozygous knock-in (KI), heterozygous KI (HE), and wild-type (WT) mice. f Diet-induced thermogenesis measured by rectal temperature after high-fat high-sucrose feeding (repeated measures ANOVA P < 0.0001) and g cold-induced thermogenesis measured by rectal temperature of mice in 4 °C condition ( n = 9:24:10; repeated measures ANOVA P = 0.29). h Isoproterenol-induced energy expenditure ( n = 4:8:4) of Aldh2 homozygous KI, HE, and WT mice. The arrow head indicates the injection time (repeated measures ANOVA P = 0.15). i Glycemic levels during the insulin sensitivity test (repeated measures ANOVA P = 0.055) and j intraperitoneal glucose tolerance tests (repeated measures ANOVA P = 0.0049), and k glycemic levels during the oral glucose tolerance test of Aldh2 KI, HE, and WT mice ( n = 49:24:42; repeated measures ANOVA P = 0.053). l Insulin levels following oral glucose load ( n = 35:14:44; repeated measures ANOVA P = 0.0048 in duplicates). Fasting serum m leptin ( n = 9:10:11; P -for-trend = 0.0002 in duplicates), n free fatty acid, and ( n = 10:10:10; P -for-trend = 0.0008 in duplicates), o adiponectin ( n = 10:10:10; P -for-trend = 0.0008 in duplicates), and p ethanol ( n = 10:10:10; P -for-trend = 0.0032 in duplicates) concentration of Aldh2 homozygous KI, HE, and WT mice on high-fat high-sucrose diet. Figure ( a ) was analyzed using the generalized linear model. Figures ( a , b , f – l ) were further analyzed using repeated measures ANOVA. Figures ( b – p ) were analyzed using tests for linear trend. All data are presented as mean and standard error (S.E.M.). The n values represent biological repeats and the number of technical repeats were expressed as duplicates or triplicates. The asterisks indicate two-sided * P < 0.05, ** P < 0.01, *** P < 0.001, **** P < 0.001. Full size image Energy expenditure is composed of resting metabolic rate, physical activity, and adaptive thermogenesis including cold-induced and diet-induced thermogenesis. Indirect calorimetry showed lower energy expenditure of Aldh2 KI and HE mice compared with WT mice. The difference is substantial during active phase (night time). Nevertheless, there is still a small but statistically difference in resting metabolic rate during inactive phase (day time) (Fig. 2a ). There was no difference of accumulative food intake measured for three weeks among three genotypes (Fig. 2b ). We also measured energy expenditure by monitoring physical activities of the mice at the age of 8–10 weeks. Daily physical activity, including wheel rotations (Fig. 2c ) and travel distances measured by HomeCage monitoring system (Fig. 2d ) were similar among the three groups. HomeCage monitoring systems did not detect significant differences in various mouse behaviors including awakening, drinking, feeding, grooming, hanging, resting, twisting, walking, and rearing up (Fig. 2e ). Consequently, we measured adaptive thermogenesis, including cold-induced, diet-induced, and isoproterenol-induced thermogenesis at the age of 8–10 weeks. For diet-induced thermogenesis, Aldh2 KI and HE mice exhibited significantly lower rectal temperature after HFHSD feeding than WT mice at the age of 20–24 weeks, indicating impaired diet-induced thermogenesis (Fig. 2f ). Compatible with rectal temperature, indirect calorimetry also revealed lower energy expenditure after diet intake of Aldh2 KI and HE mice compared with WT mice (Supplementary Fig. 2 ). For cold tolerance test, Aldh2 KI and HE mice had lower rectal temperature during 18-h prolonged cold exposure at 4 °C (Fig. 2g ) compared with WT mice at the age of 20–24 weeks. However, there was no difference of rectal temperature in 4-h acute cold tolerance test among three genotypes (Supplementary Fig. 3a ). Consistently, there was also little difference of energy expenditure in the acute cold tolerance test among three genotypes (Supplementary Fig. 3b ). Furthermore, Aldh2 KI and HE mice also have significantly lower isoproterenol-induced energy expenditure than WT mice (Fig. 2h ). However, there was no significance in serum norepinephrine among three genotypes (Supplementary Fig. 4 ). These data suggest that Aldh2 KI mice may develop obesity due to reduced energy expenditure resulting from impaired adaptive thermogenesis. Aldh2 KI mice displayed reduced insulin sensitivity and impaired glucose tolerance Since the ALDH2 Glu504Lys mutation is reported to be associated to type 2 diabetes in genome-wide association studies in East-Asians [9] , we further examined glucose homeostasis in mice. On HFHSD, insulin tolerance test (ITT)showed significantly higher blood glucose levels of Aldh2 KI and HE mice than WT mice, indicating increased insulin resistance (Fig. 2i ). Intraperitoneal glucose tolerance (i.p. GTT) showed significantly higher blood glucose levels of Aldh2 KI and HE mice than WT mice at the age of 24 weeks (Fig. 2j ). Oral glucose tolerance test (OGTT) also showed similar findings (Fig. 2k ). Aldh2 KI mice displayed a compensatory increase in insulin secretion after oral glucose load (Fig. 2l ). No differences in glucose homeostasis measured by glucose and insulin tolerance tests were found between Aldh2 KI and WT mice fed a chow diet. There were no difference in serum total cholesterols(Supplementary Fig. 5a ) and triglycerides levels (Supplementary Fig. 5b ) among three genotypes at the age of 24 weeks. However, Aldh2 KI and HE mice showed dose-dependently increase in serum leptin levels (11.13 ± 2.13 vs. 7.21 ± 0.97vs.3.24 ± 0.39 mg/ml, P -for-trend = 0.0002, Fig. 2m ), increase in free fatty acid levels (0.92 ± 0.040 vs. 1.08 ± 0.05 vs. 0.83 ± 0.05 mEq/L P -for-trend = 0.012, Fig. 2n ), decrease in serum adiponectin levels (7832.7 ± 106.4 vs. 8539.8 ± 312.4 vs. 9115.6 ± 356.9 ng/ml, P -for-trend = 0.0032 Fig. 2o ), and increase ethanol levels (0.63 ± 0.09 vs. 0.40 ± 0.06 vs. 0.34 ± 0.07 mEq/L P -for-trend = 0.0008, Fig. 2p ) compared with WT mice. Aldh2 KI mice had reduced mitochondrial fatty acid oxidation rate and lower respiratory transport chain activity in brown adipose tissue due to 4-HNE adduction In view of the reduced adaptive thermogenesis observed in the Aldh2 KI mice, we compared the expression levels of protein involved in thermogenesis including Ucp1 , Pgc1α , Prdm16, Cidea , and Dio2 between their BATs using immunoblots and real-time quantitative PCR (RT-qPCR) at the age of 24 weeks. There was no difference of these proteins between BAT isolated from Aldh2 KI and WT mice (Fig. 3a, b , Supplementary Fig. 6 ). Furthermore, there was no difference in gene expression of Ucp1 in white fat including inguinal and perigonadal fat between the Aldh2 KI and WT mice measured by RT-qPCR (Supplementary Fig. 7 ) at the age of 24 weeks. In addition, we did not observe difference in primary brown adipocyte differentiation isolated from Aldh2 KI and WT mice at the age of 4–6 weeks (Supplementary Fig. 8 ). Fig. 3: Aldh2 (acetaldehyde dehydrogenase 2) knock-in mice displayed impaired decreased fatty acid oxidation rate and mitochondrial respiration of brown adipose tissue due to increased 4-hydroxynonenal-adducted proteins. a Immunoblots and densitometry histogram showing expression of Ucp, Prdm16, Cidea, Dio2 levels ( n = 4:4) and b densitometric histogram of brown adipose tissue (BAT) from Aldh2 (wild-type) WT and (knock-in) KI mice ( P = 0.42, 0.25, 0.07, 0.74, 0.50, and 0.61 respectively). c ALDH2 enzymatic activity of recombinant WT and KI ALDH2 protein ( n = 6:6 in duplicates; P < 0.0001) and d BAT from Aldh2 WT and KI mice ( n = 9:8; P = 0.29). e 4-HNE (4-hydroxynonenal) concentration of BAT isolated from of the Aldh2 WT and KI mice ( n = 5:5; P = 0.008). f Protein carbonylation of BAT mitochondria by hydrazide biotin staining ( n = 4:4) and g immunoblots and densitometry histogram of 4-HNE-adducted mitochondrial proteins in the BAT from the Aldh2 WT and KI mice ( n = 3:3). h densitometric histogram of f and; P = 0.006 and 0.0022 respectively) ( g ). i , j 4-HNE-adducted mitochondrial proteins and amino acid residues of the BAT from the Aldh2 KI and WT mice, as identified by liquid-chromatography tandem mass spectrometry (LC-MS/MS) ( n = 2:2). k Fatty acid oxidation (FAO) rate of the whole BAT tissue isolated from the Aldh2 WT and KI mice rescued with 0.1. 0.2 and 0.4 μCi 3 H-palmitate respectively ( n = 5:7:7:7:7; P = 0.0003 and 0.0011). l FAO of primary brown adipocytes isolated from the Aldh2 WT and KI mice rescued with 0.2 and 0.6 μCi 3 H-palmitate respectively ( n = 3:3:3:4; P = 0.016). m FAO rate of induced primary brown adipocytes isolated from the WT mice treated with 0, 5, and 10 μM 4-HNE ( n = 3:3; P < 0.0001) rescued with plamitate. n Mitochondrial electron transfer chain (ETC) complex I-IV enzymatic activity isolated from the BAT of Aldh2 WT and KI mice on HFHSD ( n = 4:4; P = 0.019, 0.0018, 0.044, and 0.11 respectively). o Oxygen consumption rate (OCR) of induced primary brown adipocytes isolated from Aldh2 WT and KI mice fed on high-fat high-sucrose diet. Cells were treated with oligomycin, FCCP (carbonyl cyanide p-trifluoro methoxyphenylhydrazone), and Rotenone/Antimycin A.OCR measurements were normalized to the protein concentration. ( n = 3 per group ; repeated measures analysis of variance (ANOVA) P = 0.0026). Figures ( k – m ) were analyzed using tests for linear trend. Figures ( b – e , h , k , n , o ) were analyzed using two-sample independent t -tests. Figure ( o ) was analyzed using repeated measures ANOVA. All data are presented as mean and standard error (S.E.M.). The n values represent biological repeats and the number of technical repeats are expressed as duplicates or triplicates. The asterisks indicate two-sided * P < 0.05, ** P < 0.01, *** P < 0.001, **** P < 0.0001. Full size image ALDH2 enzymatic activity of recombinant Aldh2 KI protein is drastically reduced compared with WT proteins (Fig. 3c ). Similarly, the ex vivo ALDH2 enzymatic activity of BAT isolated from Aldh2 KI mice is also lower than those from WT mice at the age of 24 weeks (Fig. 3d ). This is accompanied with higher ex vivo 4-HNE level of BAT isolated form Aldh2 KI mice compared with WT mice (Fig. 3e ). We next examined the expression of mitochondrial respiratory complex I to V component in BAT from mice at the age of 24 weeks. These protein components are essential for the maintenance of the proton gradient in mitochondrial electron transport chain (ETC) and are required for UCP1-mediated thermogenesis. There was no difference in mitochondrial respiratory complex I to V protein components expression in the BAT of Aldh2 KI and WT mice (Supplementary Fig. 9 ). We also observed no difference in microscopic morphology of BAT, the major thermogenic organ at the age of 24 weeks (Supplementary Fig. 10 ). Since the ETC protein expression studied showed no difference between Aldh2 KI and WT mice, it implied that the decreased energy expenditure and thermogenesis were likely due to impaired protein functions. We found increased protein carbonylation (Fig. 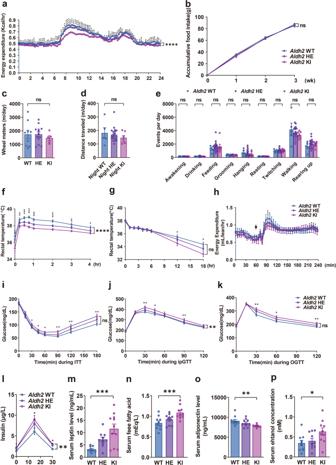Fig. 2:Aldh2(acetaldehyde dehydrogenase 2) knock-in mice mimicking human Glu504Lys mutation have reduced energy expenditure and adaptive thermogenesis. aEnergy expenditure (n= 19:27:13; repeated measures analysis of variance [ANOVA]P< 0.0001),baccumulative food intake for three weeks (n= 8:24:10; repeated measures ANOVAP= 0.70),cwheel rotations (n= 9:13:5;P-for-trend = 0.55),ddistance traveled (n= 5:20:7P-for-trend = 0.27), andebehaviors monitored by HomeCage systems (n= 5:20:7;P-for-trend = 0.88, 0.54, 0.48, 0.12, 0.31, 0.92, 0.65, 0.19, and 0.52 respectively) of theAldh2homozygous knock-in (KI), heterozygous KI (HE), and wild-type (WT) mice.fDiet-induced thermogenesis measured by rectal temperature after high-fat high-sucrose feeding (repeated measures ANOVAP< 0.0001) andgcold-induced thermogenesis measured by rectal temperature of mice in 4 °C condition (n= 9:24:10; repeated measures ANOVAP= 0.29).hIsoproterenol-induced energy expenditure (n= 4:8:4) ofAldh2homozygous KI, HE, and WT mice. The arrow head indicates the injection time (repeated measures ANOVAP= 0.15).iGlycemic levels during the insulin sensitivity test (repeated measures ANOVAP= 0.055) andjintraperitoneal glucose tolerance tests (repeated measures ANOVAP= 0.0049), andkglycemic levels during the oral glucose tolerance test ofAldh2KI, HE, and WT mice (n= 49:24:42; repeated measures ANOVAP= 0.053).lInsulin levels following oral glucose load (n= 35:14:44; repeated measures ANOVAP= 0.0048 in duplicates). Fasting serummleptin (n= 9:10:11;P-for-trend = 0.0002 in duplicates),nfree fatty acid, and (n= 10:10:10;P-for-trend = 0.0008 in duplicates),oadiponectin (n= 10:10:10;P-for-trend = 0.0008 in duplicates), andpethanol (n= 10:10:10;P-for-trend = 0.0032 in duplicates) concentration ofAldh2homozygous KI, HE, and WT mice on high-fat high-sucrose diet. Figure (a) was analyzed using the generalized linear model. Figures (a,b,f–l) were further analyzed using repeated measures ANOVA. Figures (b–p) were analyzed using tests for linear trend. All data are presented as mean and standard error (S.E.M.). The n values represent biological repeats and the number of technical repeats were expressed as duplicates or triplicates. The asterisks indicate two-sided *P< 0.05, **P< 0.01, ***P< 0.001, ****P< 0.001. 3f, h ), 4-HNE-adducted mitochondrial proteins, and 4-HNE concentration (Fig. 3g, h ) and decreased ALDH2 enzymatic activity in the BAT from the KI mice compared with WT mice at the age of 24 weeks. Using liquid-chromatography tandem mass spectrometry (LC MS/MS) analysis, we identified nineteen 4-HNE-adducted BAT mitochondrial proteins in Aldh2 KI mice and nine 4-HNE adducted mitochondrial proteins in WT mice, with eight proteins which are present in both Aldh2 KI and WT mice at the age of 24 weeks (Fig. 3 i, j). Three identified adducted sites were present in proteins involved in fatty acid oxidation (FAO) including 3-ketoacyl-CoA thiolase and propionyl-CoA carboxylase. Eleven sites were present in proteins involved in the maintenance of mitochondrial electron transport chain (ETC) including NADPH dehydrogenase (complex I), succinate dehydrogenase (complex II), cytochrome b-1 complex (complex III), ATP synthase, and glycerol-3-phoshphate dehydrogenase. Three adducted sites were present in the mitochondrial contact site and cristae organizing system (MICOS) complex, which are essential for the maintenance of inner mitochondrial membrane structure (Supplementary Table S2a ). Hence, we further evaluated the capacity of mitochondrial FAO and ETC to determine the effect of 4-HNE modification of these proteins at the age of 24 weeks. The ex vivo FAO rate of the whole BAT tissue isolated from Aldh2 KI mice was significantly decreased by 70.0% ( P < 0.001) compared with those from WT mice, which could be rescued by addition of 0.1, 0.2 and 0.4μCi 3 H-palmitate dose-dependently ( P -for-trend = 0.02) (Fig. 3k ). Consistent with the whole BAT tissue, the FAO rate of the cultured primary brown adipocytes isolated from the Aldh2 KI mice at the age of 4–6 weeks was also significantly decreased by 39.3% ( P = 0.02) compared with those from WT mice, which could be rescued by addition of 0.2 and 0.6 μCi 3 H-palmitate dose-dependently ( P -for-trend = 0.045) (Fig. 3l ). However, there was no difference of FAO in skeletal muscle and liver between KI and WT mice (Supplementary Fig. 11 ). Furthermore, addition of 4-HNE decreased FAO rate of induced primary brown adipocytes isolated from WT mice in a dose-dependent manner; FAO rates were reduced by 36% ( P < 0.01) and 60% at 5 and 10 μM 4-HNE, respectively ( P < 0.01) (Fig. 3m ). In line with the LC-MS/MS finding, we found a significant reduction in the enzymatic activity of mitochondrial respiratory complexes I, II, and III, but not complex IV, in Aldh2 KI mice compared with WT mice at the age of 24 weeks (Fig. 3n ). Oxygen consumption rate was also significantly decreased in induced primary brown adipocytes isolated from Aldh2 KI mice compared with WT mice at the age of 4 weeks (Fig. 3o ). Since FAO is the major energy source of thermogenesis and the mitochondrial ETC is essential for maintaining proton gradient required for thermogenesis, the increased protein carbonylation, especially 4-HNE-adduction may explain the impaired thermogenesis of Aldh2 KI mice. ALDH2 activator AD-9308/AD-5591 activated wild-type and mutant human ALDH2 enzymatic activity AD-9308 is a valine ester prodrug of a potent and selective small molecule ALDH2 activator AD-5591 . When administered in vivo, AD-9308 is rapidly converted to AD-5591 by esterase hydrolysis (Fig. 4a ). In vitro, AD-5591 treatment increases the catalytic activity of recombinant wild-type and mutant human ALDH2 (Fig. 4b ). 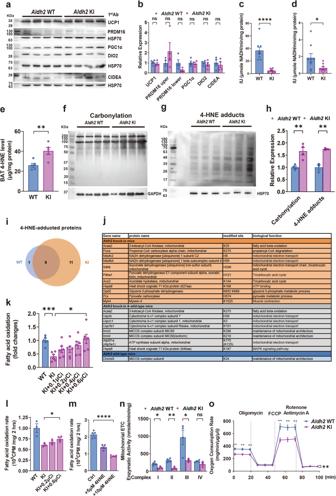Fig. 3:Aldh2(acetaldehyde dehydrogenase 2) knock-in mice displayed impaired decreased fatty acid oxidation rate and mitochondrial respiration of brown adipose tissue due to increased 4-hydroxynonenal-adducted proteins. aImmunoblots and densitometry histogram showing expression ofUcp, Prdm16, Cidea, Dio2levels (n= 4:4) andbdensitometric histogram of brown adipose tissue (BAT) fromAldh2(wild-type) WT and (knock-in) KI mice (P= 0.42, 0.25, 0.07, 0.74, 0.50, and 0.61 respectively).cALDH2 enzymatic activity of recombinant WT and KI ALDH2 protein (n= 6:6 in duplicates;P< 0.0001) anddBAT fromAldh2WT and KI mice (n= 9:8;P= 0.29).e4-HNE (4-hydroxynonenal) concentration of BAT isolated from of theAldh2WT and KI mice (n= 5:5;P= 0.008).fProtein carbonylation of BAT mitochondria by hydrazide biotin staining (n= 4:4) andgimmunoblots and densitometry histogram of 4-HNE-adducted mitochondrial proteins in the BAT from theAldh2WT and KI mice (n= 3:3).hdensitometric histogram offand;P= 0.006 and 0.0022 respectively) (g).i,j4-HNE-adducted mitochondrial proteins and amino acid residues of the BAT from theAldh2KI and WT mice, as identified by liquid-chromatography tandem mass spectrometry (LC-MS/MS) (n= 2:2).kFatty acid oxidation (FAO) rate of the whole BAT tissue isolated from theAldh2WT and KI mice rescued with 0.1. 0.2 and 0.4 μCi3H-palmitate respectively (n= 5:7:7:7:7;P= 0.0003 and 0.0011).lFAO of primary brown adipocytes isolated from theAldh2WT and KI mice rescued with 0.2 and 0.6 μCi3H-palmitate respectively (n= 3:3:3:4;P= 0.016).mFAO rate of induced primary brown adipocytes isolated from the WT mice treated with 0, 5, and 10 μM 4-HNE (n= 3:3;P< 0.0001) rescued with plamitate.nMitochondrial electron transfer chain (ETC) complex I-IV enzymatic activity isolated from the BAT ofAldh2WT and KI mice on HFHSD (n= 4:4;P= 0.019, 0.0018, 0.044, and 0.11 respectively).oOxygen consumption rate (OCR) of induced primary brown adipocytes isolated fromAldh2WT and KI mice fed on high-fat high-sucrose diet. Cells were treated with oligomycin, FCCP (carbonyl cyanide p-trifluoro methoxyphenylhydrazone), and Rotenone/Antimycin A.OCR measurements were normalized to the protein concentration. (n= 3 per group;repeated measures analysis of variance (ANOVA)P= 0.0026). Figures (k–m) were analyzed using tests for linear trend. Figures (b–e,h,k,n,o) were analyzed using two-sample independentt-tests. Figure (o) was analyzed using repeated measures ANOVA. All data are presented as mean and standard error (S.E.M.). The n values represent biological repeats and the number of technical repeats are expressed as duplicates or triplicates. The asterisks indicate two-sided *P< 0.05, **P< 0.01, ***P< 0.001, ****P< 0.0001. In vivo, AD-9308 administration showed a favorable pharmacokinetic profile in mice when administered orally or intravenously with high bioavailability (Supplementary Table 3 ). Fig. 4: ALDH2 (Acetaldehyde Dehydrogenase 2) activator AD-9308 enhanced ALDH2 enzymatic activities. a Prodrug AD-9308 is converted to AD-5591 by esterase hydrolysis in vivo. b AD-5591 (100 μM) or alda-1 (100 μM) significantly increases the enzymatic activity of recombinant WT and mutant human ALDH2 proteins ( n = 3 per group in duplicates, left panel: one-way analysis of variance (ANOVA) P < 0.0001, Tukey’s post hoc test: column 1 vs. 2: P = 0.04, column 1 vs. 3: P < 0.001, and column 2 vs. 3. P < 0.001, right panel: one-way ANOVA P < 0.0001, Tukey’s post hoc test: column 1 vs. 2: P = 0.0056, column 1 vs. 3: P = 0.0006, and column 2 vs. 3. P < 0.001). c Ribbon diagram showing the binding pocket of AD-5591 within human WT ALDH2. d LigPlot (Ligand-Protein Interaction Diagrams) showing the bonds between AD-5591 and human WT ALDH2. e Regional ribbon diagram showing the binding of AD-5591 and NAD + with WT ALDH2. Figure ( b ) was analyzed by one-way ANOVA with Tukey’s post-hoc tests. All data are presented as mean and standard error (S.E.M.). The n values represent biological repeats and the number of technical repeats were expressed as duplicates or triplicates. The asterisks indicate two-sided * P < 0.05, ** P < 0.01, *** P < 0.001. Full size image Alda-1 allosterically activates ALDH2 mainly by partially blocking the substrate exit tunnel, thereby accelerating the substrate-enzyme collision without impeding the catalytic sites of Cys302 and Glu268; [26] Alda-1 also inhibits substrate-induced ALDH2 inactivation by protecting Cys301 and Cys303 oxidation [25] , [30] . Using molecular docking, we found that the binding pocket for AD-5591 (Fig. 4c ) is close to that of Alda-1 (Supplementary Fig. 12a ). Similar to Alda-1 (Supplementary Fig. 12b ), AD-5591 is bound within a hydrophobic collar by Tyr456, Val458, Lys127, Met124, Gln462, Gly460, Phe459, Val120, and Phe292 of human ALDH2 (Fig. 4d ). This binding site leaves the catalytic sites Cys302 and Glu268 unimpeded ( Fig. 4e , Supplementary Fig. 12c ). Therefore, the mechanism by which AD-5591 activates ALDH2 is very similar to Alda-1 . Furthermore, Alda-1 forms a single hydrogen bond with the Asp457 residue of ALDH2. Yet, in our modeling analyses, AD-5591 forms one additional hydrogen bond with Ala461 (Fig. 4e ), which may explain its higher affinity to ALDH2 than Alda-1 . ALDH2 activator AD-9308/AD-5591 lowered 4-HNE and attenuated diet-induced obesity, fatty liver, insulin resistance, and glucose intolerance in both WT and Aldh2 KI mice In view of the marked reduction in Aldh2 expression in diet-induced obese mice (Supplementary Fig. 13 ), we next explored whether Aldh2 activation can rescue these obesity-associated phenotypes. From the age of 10 weeks when HFHSD was started, Aldh2 KI and WT mice were treated with vehicle, 20 mg/kg/day or 60 mg/kg/day of AD-9308 by oral gavage for 20 weeks (Fig. 5a ). As shown in Fig. 5 b–e, AD-9308 treatment effectively reduced the diet-induced weight gain in both Aldh2 KI and WT mice. Weight of perigonadal fat, inguinal fat, omental fat decreased with AD-9308 treatment dose-dependently (Fig. 5 e–h) with reduced diet-induced adipocyte hypertrophy (Fig. 5i ). AD-9308 treatment reduced the extent of hepatic steatosis (Fig. 5 j, k, l) and the levels of hepatic triglycerides contents in both Aldh2 KI and WT mice in a dose-dependent manner (Fig. 5m ). Fig. 5: ALDH2 (Acetaldehyde Dehydrogenase 2) activator AD-9308 treatment prevented diet-induced obesity and fatty liver. a Study flow of AD-9308 treatment. Body weight of b Aldh2 wild-type (WT) and c knock-in (KI) mice treated with vehicle, low-dose AD-9308 (20 mg/kg/day), and high-dose AD-9308 (60 mg/kg/day) (repeated measures analysis of variance [ANOVA] P = 0.0051 and P < 0.0001). d Gross appearance of the mice and e perigonadal fat of Aldh2 WT and KI mice treated with AD-9308 . Weight of f perigonadal fat ( P -for-trend = 0.0048 and 0.0043), g inguinal fat ( P -for-trend = 0.003 and 0.01), and h omental fat ( P -for-trend = 0.0023 and 0.0024) of the Aldh2 WT and KI mice treated with AD-9308 . i H&E (hematoxylin and eosin) stain of perigonadal fat. The scale bar of is 100 µm. j Gross appearance and k weight of liver of Aldh2 WT and KI mice treated with AD-9308 ( P -for-trend = 0.06 and 0.0032). l H&E stain of liver and m hepatic triglycerides (TG) content of the Aldh2 WT and KI mice treated with AD-9308 on high-fat high-sucrose diet ( n = 11:14 for the vehicle group; n = 12:15 for 20 mg/kg/day group; n = 9:12 for 60 mg/kg/day group in duplicates; P -for-trend = 0.039 and 0.0004). The scale bar of is 100 µm. Figures ( b and c ) were analyzed using repeated-measures ANOVA. Figures ( f – h , k , and m ) were analyzed using were analyzed using tests for linear trends. All data are presented as mean and standard error (S.E.M.). The n values represent biological repeats and the number of technical repeats were expressed as duplicates or triplicates. The asterisks indicate two-sided * P < 0.05, ** P < 0.01, *** P < 0.001, **** P < 0.001. Full size image Fasting glucose levels were lowered by AD-9308 treatment in both Aldh2 WT and KI mice (Fig. 6 a, b). AD-9308 treatment effectively reduced insulin resistance in both WT (Fig. 6c ) and KI (Fig. 6d ) mice and significantly improved glucose tolerance of both WT (Fig. 6e ) and KI (Fig. 6f ) mice in a dose-dependent manner. AD-9308 also decreased serum 4-HNE levels in both mice groups dose-dependently (Fig. 6g ) at the age of 30 weeks. Figure 6h shows the summary diagram depicting how reducing 4-HNE by ALDH2 activator AD-9308 ameliorates metabolic disturbances. Fig. 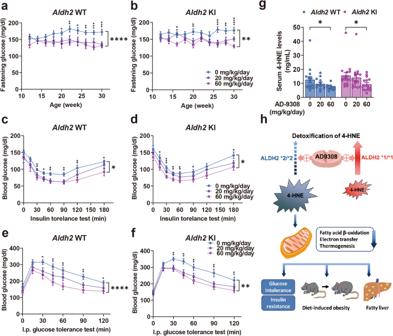Fig. 6: ALDH2 activator AD-9308 treatment ameliorated diet-induced insulin resistance and glucose intolerance. Fasting glucose level of theaAldh2wild-type(WT) andbknock-in (KI) mice treated with vehicle, low-doseAD-9308(20 mg/kg/day), and high-doseAD-9308(60 mg/kg/day) (repeated measures analysis of variance [ANOVA]P< 0.0001 and 0.0016).c,dGlycemic levels during the insulin sensitivity test (repeated measures ANOVAP= 0.014 and 0.012) ande,fintraperitoneal glucose tolerance test of theAldh2WT and KI mice treated withAD-9308(n= 15:15 for the vehicle group;n= 14:16 for 20 mg/kg/day group;n= 9:14 for 60 mg/kg/day group; repeated measures ANOVAP< 0.0001 and 0.0039).gSerum 4-HNE (4-hydroxynonenal) levels of theAldh2WT and KI mice treated withAD-9308(n= 15:16 for the vehicle group;n= 12:14 for 20 mg/kg/day group;n= 12:14 for 60 mg/kg/day group in duplicates; P-for-trend = 0.025 and 0.044) on high-fat high-sucrose diet.hSummary diagram depicting how reducing 4-HNE byAD-9308ameliorates metabolic disturbances. Figures (a–g) were analyzed using tests for linear trends. Figures (a–e) were further analyzed using repeated measures ANOVA. All data are presented as mean and standard error (S.E.M.). Thenvalues represent biological repeats and the number of technical repeats were expressed as duplicates or triplicates. The asterisks indicate two-sided *P< 0.05, **P< 0.01, ***P< 0.001, ****P< 0.001. 6: ALDH2 activator AD-9308 treatment ameliorated diet-induced insulin resistance and glucose intolerance. Fasting glucose level of the a Aldh2 wild-type(WT) and b knock-in (KI) mice treated with vehicle, low-dose AD-9308 (20 mg/kg/day), and high-dose AD-9308 (60 mg/kg/day) (repeated measures analysis of variance [ANOVA] P < 0.0001 and 0.0016). c , d Glycemic levels during the insulin sensitivity test (repeated measures ANOVA P = 0.014 and 0.012) and e , f intraperitoneal glucose tolerance test of the Aldh2 WT and KI mice treated with AD-9308 ( n = 15:15 for the vehicle group; n = 14:16 for 20 mg/kg/day group; n = 9:14 for 60 mg/kg/day group; repeated measures ANOVA P < 0.0001 and 0.0039). g Serum 4-HNE (4-hydroxynonenal) levels of the Aldh2 WT and KI mice treated with AD-9308 ( n = 15:16 for the vehicle group; n = 12:14 for 20 mg/kg/day group; n = 12:14 for 60 mg/kg/day group in duplicates; P-for-trend = 0.025 and 0.044) on high-fat high-sucrose diet. h Summary diagram depicting how reducing 4-HNE by AD-9308 ameliorates metabolic disturbances. Figures ( a – g ) were analyzed using tests for linear trends. Figures ( a – e ) were further analyzed using repeated measures ANOVA. All data are presented as mean and standard error (S.E.M.). The n values represent biological repeats and the number of technical repeats were expressed as duplicates or triplicates. 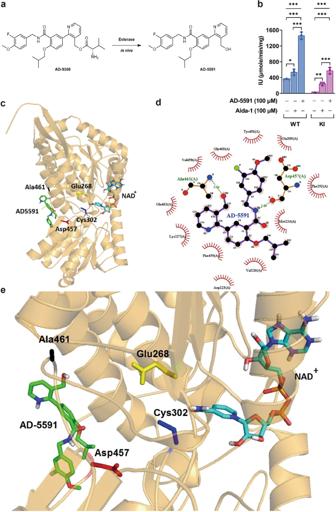The asterisks indicate two-sided * P < 0.05, ** P < 0.01, *** P < 0.001, **** P < 0.001. 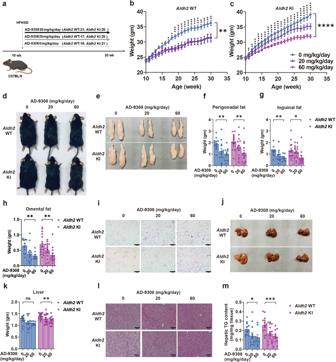Fig. 4: ALDH2 (Acetaldehyde Dehydrogenase 2) activator AD-9308 enhanced ALDH2 enzymatic activities. aProdrugAD-9308is converted toAD-5591by esterase hydrolysis in vivo.bAD-5591(100 μM) oralda-1(100 μM) significantly increases the enzymatic activity of recombinant WT and mutant human ALDH2 proteins (n= 3 per group in duplicates, left panel: one-way analysis of variance (ANOVA)P< 0.0001, Tukey’s post hoc test: column 1 vs. 2:P= 0.04, column 1 vs. 3:P< 0.001, and column 2 vs. 3.P< 0.001, right panel: one-way ANOVAP< 0.0001, Tukey’s post hoc test: column 1 vs. 2:P= 0.0056, column 1 vs. 3:P= 0.0006, and column 2 vs. 3.P< 0.001).cRibbon diagram showing the binding pocket ofAD-5591within human WT ALDH2.dLigPlot (Ligand-Protein Interaction Diagrams) showing the bonds betweenAD-5591and human WT ALDH2.eRegional ribbon diagram showing the binding ofAD-5591and NAD+with WT ALDH2. Figure (b) was analyzed by one-way ANOVA with Tukey’s post-hoc tests. All data are presented as mean and standard error (S.E.M.). Thenvalues represent biological repeats and the number of technical repeats were expressed as duplicates or triplicates. The asterisks indicate two-sided *P< 0.05, **P< 0.01, ***P< 0.001. Fig. 5: ALDH2 (Acetaldehyde Dehydrogenase 2) activator AD-9308 treatment prevented diet-induced obesity and fatty liver. aStudy flow ofAD-9308treatment. Body weight ofbAldh2wild-type (WT) andcknock-in (KI) mice treated with vehicle, low-doseAD-9308(20 mg/kg/day), and high-doseAD-9308(60 mg/kg/day) (repeated measures analysis of variance [ANOVA]P= 0.0051 andP< 0.0001).dGross appearance of the mice andeperigonadal fat ofAldh2WT and KI mice treated withAD-9308. Weight offperigonadal fat (P-for-trend = 0.0048 and 0.0043),ginguinal fat (P-for-trend = 0.003 and 0.01), andhomental fat (P-for-trend = 0.0023 and 0.0024) of theAldh2WT and KI mice treated withAD-9308.iH&E (hematoxylin and eosin) stain of perigonadal fat. The scale bar of is 100 µm.jGross appearance andkweight of liver ofAldh2WT and KI mice treated withAD-9308(P-for-trend = 0.06 and 0.0032).lH&E stain of liver andmhepatic triglycerides (TG) content of theAldh2WT and KI mice treated withAD-9308on high-fat high-sucrose diet (n= 11:14 for the vehicle group;n= 12:15 for 20 mg/kg/day group;n= 9:12 for 60 mg/kg/day group in duplicates;P-for-trend = 0.039 and 0.0004). The scale bar of is 100 µm. Figures (bandc) were analyzed using repeated-measures ANOVA. Figures (f–h,k, andm) were analyzed using were analyzed using tests for linear trends. All data are presented as mean and standard error (S.E.M.). Thenvalues represent biological repeats and the number of technical repeats were expressed as duplicates or triplicates. The asterisks indicate two-sided *P< 0.05, **P< 0.01, ***P< 0.001, ****P< 0.001. Full size image Pathological examination revealed no abnormalities in liver or kidney in both Aldh2 WT and KI mice treated with AD-9308 for 20 weeks (Supplementary Table 4 ). Serum alanine aminotransferase (ALT) and creatinine levels were also not different between groups after AD-9308 treatment for 20 weeks (Supplementary Fig. 14 ). Finally, to identify 4-HNE-adducted proteins modified by AD-9308 treatment, we performed LC-MS/MS analyses of the BAT isolated from Aldh2 WT and KI mice treated or not treated with AD-9308 at the age of 30 weeks. As shown in Supplementary Fig. 15a and Supplementary Table S2b , treatment of AD-9308 reduced the number of 4-NHE-adducted proteins in the BAT from Aldh2 WT mice from fourteen to four. Among these ten proteins, eight proteins are involved in mitochondrial ETC and FAO including the Trifunctional enzyme subunit alpha, mitochondrial (Hadha), Succinate dehydrogenase [ubiquinone] flavoprotein subunit, mitochondrial (Sdha), Cytochrome b-c1 complex subunit 1, mitochondrialUqcrc1, Long-chain-fatty-acid--CoA ligase(Acsl1), Trifunctional enzyme subunit beta, mitochondrial(Hadhb), 3-ketoacyl-CoA thiolase, mitochondrial (Acaa2), Cytochrome b-c1 complex subunit 7 (Uqcrb), and Cytochrome c oxidase subunit 6C (Cox6c) being eliminated by AD9308 (Supplementary Fig. 15b ). Similarly, treatment of AD-9308 reduced the number of 4-NHE-adducted proteins in the BAT from Aldh2 KI mice from eighteen to four (Supplementary Fig. 16a ). Among these fourteen proteins, twelve proteins are involved in mitochondrial ETC and FAO including the Trifunctional enzyme subunit alpha, mitochondrial (Hadha), Succinate dehydrogenase [ubiquinone] flavoprotein subunit, mitochondrial (Sdha), Cytochrome b-c1 complex subunit 1, mitochondrial (Uqcrc1), Cytochrome b-c1 complex subunit 2, mitochondrial (Uqcrc2), Trifunctional enzyme subunit beta, mitochondrial (Hadhb), Cytochrome c oxidase subunit NDUFA4 (Ndufa4), Mitochondrial carnitine/acylcarnitine carrier protein (Slc25a20), Cytochrome b-c1 complex subunit 7 (Uqcrb), NADH dehydrogenase [ubiquinone] 1 beta subcomplex subunit 10 (Ndufb10), NADH dehydrogenase [ubiquinone] iron-sulfur protein 6, mitochondrial (Ndufs6), and Cytochrome c oxidase subunit 6C(Cox6c) being eliminated by AD-9308 (Supplementary Fig. 16b and Supplementary Table S2c ). These results were consistent with the results comparing 4-HNE-adduced proteins of BAT between Aldh2 WT and KI mice, showing ALDH2 modulates mitochondrial ETC and FAO function in BAT. The prevalence of obesity and diabetes mellitus has surged in the past decades and is predicted to continue to rise, especially in East and South Asia [1] . This trend is largely caused by high-calorie diet enriched in fat and sugar, sedentary lifestyle, and their interaction with genetic predisposition [1] , [2] . Genome-wide association studies have confirmed many genetic loci associated type 2 diabetes and obesity. Specifically, several genetic loci are East Asian-specific. Genetic variants in or near the CDKAL1 , KLF9 , GP2 , ALDH2 , and ITIH4 genes are associated with obesity [32] , [33] and genetic variants in or near the GDAP1 , PTF1A , SIX3 , ALDH2 , and PAX4 genes [9] , [34] are specifically associated with type 2 diabetes in East Asians. Among them, the ALDH2 Glu504Lys mutation that affects 560 million East Asians or nearly 8% of global population is associated with body mass index, type 2 diabetes, and serum lipids in large meta-analyses of genome-wide association studies. We demonstrated that Aldh2 KI mice carrying the East Asian-specific Glu504Lys mutation were more prone to develop diet-induced obesity, fatty liver, insulin resistance and glucose intolerance than WT mice Importantly, the ALDH2 activator AD-9308 increased both the catalytic activity of WT and mutant enzyme, reduced serum 4-HNE levels, and effectively alleviated diet-induced obesity, fatty liver, insulin resistance, and glucose intolerance in both Aldh2 KI and WT mice in a dose-dependent manner. BAT is a highly specialized organ enriched in Ucp1 for adaptive thermogenesis. Although Aldh2 KI mice exhibited impaired thermogenesis, unexpectedly, they did not have altered Ucp1 or associated thermogenesis gene expression. Instead, we found that the ALDH2 enzymatic activity is reduced and the 4-HNE level is increased in the BAT from Aldh2 KI mice. Proteomics screening found that several key mitochondrial proteins involved in mitochondrial fatty acid oxidation (FAO) and electron transfer chain (ETC) were modified by 4-HNE adduction, leading to markedly (~70%) reduced FAO and mitochondrial respiration. Consistently, previous studies have shown that 4-HNE is mainly generated from oxidation of mitochondrial membranes, with 30% of 4-HNE-adducted proteins located within mitochondria [35] , [36] . We further found the serum free fatty acid level is increased and the respiratory exchange rate (RER) measured by indirect calorimetry is increased in Aldh2 KI mice, further indicating impaired fatty acid utilization. Mitochondrial FAO and ETC are required for the maintenance of the proton gradient in the inter-membranous space, which is essential for Ucp1-mediated adaptive thermogenesis. In our study, we found that the thermogenic capacity of Aldh2 KI mice was reduced. Fatty acids serve as the main fuel suppliers for thermogenesis [37] . It has been estimated that fatty acids in the BAT contribute 74–84% of the fuel for thermogenesis [37] . Cpt1 is the rate-limiting enzyme for the translocation of fatty acids into mitochondria for β-oxidation. Cpt1b +/− mice developed fatal hypothermia following cold challenge [38] . Adipose-specific Cpt2 -knockout mice presented a hypothermic phenotype when exposed to cold [39] . Mice deficient in fatty acid β-oxidation enzymes, including very-long-chain acyl-CoA dehydrogenase (VLCAD), long-chain acyl CoA dehydrogenase (LCAD), and short-chain acyl CoA dehydrogenase (SCAD) also displayed cold intolerance [40] , [41] , [42] . These data indicate that mitochondrial FAO is critical for adaptive thermogenesis. Furthermore, BAT-specific Lkb1 -knockout mice, which have reduced expression of ETC complex proteins, also developed impaired thermogenesis [43] , indicating that the integrity of mitochondrial ETC machinery is essential for adaptive thermogenesis. These data strongly support our findings that 4-HNE adduction to mitochondrial proteins involved in mitochondrial FAO and ETC could lead to impaired adaptive thermogenesis. Collectively, these data indicate that the significantly reduced Aldh2 activity of Aldh2 KI mice results in elevated toxic aldehydes levels and, especially 4-HNE and increased 4-HNE adduction to proteins involved in mitochondrial reduced FAO and mitochondrial respiration of BAT, leading to markedly decreased FAO rate and mitochondrial respiration and subsequent reduced adaptive thermogenesis and energy expenditure. The reduced thermogenesis and energy expenditure result in die-induced obesity and associated metabolic disorders including fatty liver, insulin resistance, and glucose intolerance. On the contrary, over-expression of Aldh2 has been shown to decrease both the heart and liver weight and mitochondrial injury in mice fed on a high-fat diet [44] . ALDH2 metabolizes bioactive toxic aldehydes by oxidation. In addition to ALDH2, one of the major pathways to detoxify 4-HNE is mediated through glutathione transferases (GSTs) by conjugation to glutathione. Gsta4 is one of the isoforms of GST with the highest conjugation activity for 4-HNE. Consistent with the present finding, disruption of Gsta4 in mice increased 4-HNE levels and caused obesity in mice [45] . Disruption of the Gst-10 gene, which causes a 50% increase in 4-HNE adducts in C.elegans also resulted in fat accumulation and direct treatment with 4-HNE increases lipid storage in C.elegans [46] . Conversely, over-expression of Gst-10 led to 4-HNE reduction and a lean phenotype [46] . Glutathione peroxidase 4 ( Gpx4 ), which resides in the inner mitochondrial membrane, is a scavenger that reduces lipid peroxides. Deficiency of Gpx4 in mice increased the number of 4-HNE adducts and exacerbated glucose intolerance, dyslipidemia, and fatty liver [47] . Our study also showed that the Aldh2 KI mice had more severe hepatic steatosis than the WT mice when fed on HFHSD, which can be reversed by AD-9308 treatment. In line with the present results, Alda-1 , a prototype of the ALDH2 activator has been shown to alleviate nonalcoholic hepatic steatosis in apolipoprotein E-knockout mice [48] and reversed alcohol-induced hepatic steatosis in animals [49] , supporting activation of ALDH2 also prevents both alcohol and non-alcoholic hepatic steatosis. Our study has several limitations. First, obesity and related metabolic phenotypes in the Aldh2 KI mice were observed only when fed on HFHSD and not when placed on chow diet, the metabolic phenotypes were not different between the Aldh2 KI and WT mice. Therefore, our findings may not be generalized to the entire population. The HFHSD for mice consists of 58% calories from fat and 12% calories from sucrose; while the chow diet is composed of 13% calories from fat and 3% calorie from sucrose. According to the Nutrition and Health Surveys in Taiwan (NAHSIT) in 2008, the average calorie intake from fat and sucrose is 33% and 8% in adults in Taiwan [50] . In the National Health and Nutrition Examination Survey of U.S. adults, the average calorie intake from fat and sucrose is 35% and 14% in 2012 [51] , [52] . The sucrose content is comparable between HFHSD for mice and modern human diet but the fat content of HFHSD is higher than human diet. Even if this concern is relevant, the findings of this study are still substantial given the large number of East Asians (560 million people) carrying this inactivating mutation (Glu504Lys) in the ALDH2 gene. Second, although the metabolic disorders were normalized in mice treated with AD-9308 for 5 months without pathological changes in the liver and kidney, long-term safety should be formally determined with GLP standard. Last, humans and other mammals have 19 different aldehyde dehydrogenases (ALDH) and at least six are found in the mitochondria [7] . Although AD-9308 does not activate ALDH1A1, ALDH3A1, ALDH4A1, ALDH5A1 and ALDH7A1 members of the ALDH family, it is possible that AD-9308 may still have non-specific effect on other ALDHs. Our study has important clinical implications. We showed that reduced activity of the mitochondrial enzyme, ALDH2, exacerbates obesity-associated pathologies. These pathologies correlate with increased aldehydic load and inactivation of critical mitochondrial proteins involved in FAO and ETC. Significantly, we showed that treatment with an activator of ALDH2, such as AD-9308 prevented these pathologies. These data provide strong evidence for a critical role of toxic aldehydes accumulation and defective ALDH2 activity in the pathogenesis of obesity, diabetes, and fatty liver disease. Our study provides a feasible strategy by targeting ALDH2 for the treatment of obesity-associated metabolic disorders which are rising rapidly in human populations, particularly in the East and South Asia. Animal experiments, administration of diets and drug treatment All animal experiments were performed according to institutional ethical guidelines and were approved by the Institutional Animal Care and Use Committee (IACUC) (IACUC Approval No: 20110418) of the National Taiwan University College of Medicine and College of Public Health, which is accredited by the Association for Assessment and Accreditation of Laboratory Animal Care International (AAALAC). Aldh2 KI mice with C57BL6/J background are kind gifts from Dr. Daria Mochly-Rosen of the Stanford University (Supplementary Fig. 17 ) and AD-9308 is a kind gift from Dr. Wenjin Yang from the Foresee Pharmaceuticals, Co., Ltd. The mice were housed at 22–24 °C with light: dark cycles of 12:12 h. The mice were fed either a HFHSD (cat. no. D12331, Research Diets) which provided 58% kilocalorie from fat and 12.5% kilocalorie from sucrose or a chow diet (cat no. 5001, Lab Diet). Mice were bred by mating heterozygous mating. For the animal experiments, AD-9308 was dissolved in water and was delivered daily to mice by oral gavage. Only male mice were used in this study. Mice were anesthetized using inhaled 1.5–2.0% isoflurane (NDC 66794-017-25, Piramal) at a flow rate of 2 liter/min. Glucose and insulin tolerance test Oral and intraperitoneal GTT were evaluated after 6 h of fasting at the age of 24 weeks. Tail blood glucose was collected at 0, 15, 30, 45, 60, 90, and 120 min after oral gavage or intraperitoneal injection of glucose water (1 g/kg) and measured by a glucometer (ACCU-CHECK Performa, Roche). For the ITT, mice were intraperitoneally injected 1 U/kg insulin (Humulin R, Eli Lilly) after 4 h of fasting. Tail blood was collected at 0, 15, 30, 45, 60, 90, 120, and 180 min after injection. Energy expenditure, food intake, physical activity, and animal behavior Metabolic measurements (food and water intake, locomotor activity, VO 2 consumption and VCO 2 . production) were obtained using the Columbus Instruments’ Comprehensive Lab Animal Monitoring System. (CLAMS-HC)at the age of 8 weeks. Monitoring was performed for 3 days after mice have been acclimatized to the cages for 3 days. Animal behavior including awakening, drinking, feeding, grooming, hanging, resting, twisting, walking, and rearing up were recorded by the Clever HomeCage Scan system 3.0 for 24 h after acclimation for 3 days. Accumulative diet intake was measured by weighting diet consumed by two mice of the same genotype in their home cage weekly for 3 weeks. Body composition analysis Body composition was analyzed using the Bruker minispec Live Mice Analyzer (LF50) based on time domain nuclear magnetic resonance technology (TD-NMR) at the age of 24 weeks. The tissue contrast is high between fat and muscle based on relative relaxation times. It acquires and analyzes TD-NMR signals from all protons in the entire sample volume and can provide fat, free and total fluid and lean tissue values for whole-body composition of live, un-anesthetized mice. The measure frequency is 7.5 Hertz. The accuracy is within 1 % and each measurement was performed in triplicates. Isoproterenol-induced energy expenditure Isoproterenol (20 mg/kg) was dissolved in normal saline with 1:100 dilution (1 mg/100 μL) at the age of 8–10 weeks. After single injection subcutaneously over the neck, energy expenditure was recorded for 5 h. Hepatic triglycerides content measurement Approximately 80 mg of liver tissue from mice at the age of 24 weeks was homogenized in 1800 μl of chloroform/methanol (2:1). Then, 360 μl of H 2 O was added. The homogenates were centrifuged and the lower 200-μl layer was added with 100 μlof chloroform with 4% Triton X-100 and then dried in a chemical hood. The dried pellet was re-dissolved with 200 μl of H 2 O for determination of triglyceride concentrations with Wako TG LabAssay kit (cat. no. 290-63701, Wako). Cold tolerance test and diet-induced thermogenesis test For the acute cold tolerance test, 20–24-week-old mice with matched body weight from the two groups were placed individually on HFHSD in a 4 °C chamber for 4 h without food supply. For prolonged cold tolerance test, the rectal temperature of the mice was measured after 0, 1, 2, 3, 4, 5, 6, 12, and 18 h a 4 °C chamber with food and water supply. For the diet-induced thermogenesis test, 24-week-old mice were fasted overnight for 18 h. Then, their rectal temperature was measured at 0, 15, 30, 60, 120, 180, and 240 min after HFHSD re-feeding. Real-time quantitative PCR (RT-qPCR) RT-qPCR was performed using SYBR green reagent (cat. no. 11203ES08, YEASEN). The primer sequences for mouse Ucp1 and Ppia is list in Supplementary Table S1 . RT-qPCR reactions were performed using an ABI 7900HT FAST (Applied Biosystems). All qPCR reactions were run in duplicate for each sample. Primary brown adipocyte culture BAT from Aldh2 WT and KI mice aged 4–6 weeks was minced and digested by type I collagenase (cat. no. 17018029, Thermo Fisher Scientific) in HEPES buffer. The stromal vascular fraction (SVF) was obtained by centrifugation and cultured in Dulbecco’s modified Eagle medium: nutrient mixture F-12 (DMEM/F-12) (cat. no. 12500062, HyClone) supplemented with 10% FBS (cat. no. 04-001-1A, Biological Industries) and 1× antibiotic/antimycotic solution (cat. no. SV30079.01, HyClone). For cell differentiation, preadipocytes were cultured in differentiation medium containing 10% FBS, 0.5 mM isobutyl-methylxanthine, 1 μg/ml insulin, 5 μM dexamethasone, 1 nM T3, and 125 μM indomethacin for 2 days. Next, cells were maintained in the medium containing DMEM/F12 with 10% FBS, 1 μg/ml insulin, and 1 nM T3. The medium was changed every 2 days. Isolation of mitochondria from brown adipose tissue For fatty acid assay, BAT was taken from Aldh2 WT or KI mice fed a HFHSD for 5 weeks. Isolation of mitochondria was performed according to published protocols [53] . Briefly, BAT was homogenized in 10% w/v of ice-cold STE buffer (0.25 M sucrose, 1 mM EDTA, 10 mM Tris-HCl, pH7.4) by 10 strokes of the loose-fitting pestle of the Dounce homogenizer. The homogenate was spun at 500 × g and 4 °C for 10 min, and the supernatant was kept as the mitochondrial sample for FAO. Fatty acid oxidation (FAO) assay FAO measurements were performed using labeled 3 H-palmitic acid and 3 H 2 O production was assessed as previously described [54] . Briefly, for FAO rate of differentiated primary cells, the capture of 3 H 2 O was measured after a 2-h incubation with 5 mM palmitate/BSA buffer including 0.5 μCi [ 3 H]-palmitate (cat. no. PK-NET043001MC, PerkinElmer) in the presence of 1 mM carnitine. For FAO rate rescued assay of differentiated primary cells, the capture of 3 H 2 O was measured after a 2-h incubation with 5 mM palmitate/BSA buffer including a concentration gradient, 0.5, 0.7 and 1.1 μCi [ 3 H]-palmitate (cat. no. PK-NET043001MC, PerkinElmer) in the presence of 1 mM carnitine. For FAO rate of whole BAT, the isolated mitochondria were placed in a 24-well plate and added incubated with reaction buffer (100 mM sucrose, 10 mM Tris-HCl, 5 mM KH 2 PO 4 , 0.2 mM EDTA, 80 mM KCl, 1 mM MgCl 2 , 2 mM L-carnitine, 0.1 mM malate, 0.05 mM coenzyme A, 2 mM ATP, 1 mM dithiothreitol, and 7% BSA/500 μM palmitate/0.01 μCi/μl [ 3 H]-palmitate) at 37 °C for 60 min. For FAO rate rescued assay of whole BAT, the mitochondria were tested in the same condition as above mention, expect the palmitate concentration was used as a concentration gradient, 0.01, 0.01125, 0.0125 and 0.015 μCi/μl. 3 H 2 O was isolated by oil-water separation with chloroform, methanol and KCl/HCl. The average counts per minute (CPM) were measured using a liquid scintillation counter. Biotin hydrazide staining for carbonylated protein For detection of carbonylated protein, samples were chemically reduced by NaBH 4 and then incubated with 0.5 mM EZ-link biotin hydrazide (cat. no.21339, Pierce) for 1 h. After coupling, the samples were separated by 10% SDS-PAGE (sodium dodecyl sulfate polyacrylamide gel electrophoresis gel) and transferred to PVDF (polyvinylidene fluoride) membrane. The membrane was blocked with 10% skim milk in PBS containing 0.05% Tween-20 (PBST) at 4 °C overnight and then incubated with streptavidin-HRP (horseradish peroxidase) (1:1000, cat no. 890803, BD Biosciences) for 1 h at room temperature. Chemiluminescence signals were developed with HRP substrate (cat. no. WBLUR0500, Millipore). Plasmid construction, expression and purification of human ALDH2 in Escherichia coli E. coli BL21 (DE3) (cat no. EC0114, Thermo Scientific) was transformed with pTrcHi-WT ALDH2 and pTrcHi-KI ALDH2 [29] . The transformants were cultured and then induced to express recombinant proteins using 0.4 mM IPTG for 16–18 h at 25 °C. The cells were harvested by centrifugation and broken in lysis buffer by sonication on ice. The recombinant ALDH2 protein was purified with NI-NTA resin (cat. no. 88222, Thermo Fisher) following the user manual. ALDH2 enzymatic activity assays ALDH2 activity was measured by monitoring the production rate of NADH (nicotinamide adenine dinucleotide)/min at 340 nm and 25 °C. Enzyme activity was assayed in 100 μl of reaction mixtures containing 50 mM Na 4 P 2 O 7 (pH 9.5), 0.01% BSA, 10 mM NAD + , 50 μM acetaldehyde and recombinant ALDH2 with or without 100 μM AD-5591 or Alda-1 . One enzymatic activity unit was defined as the production of 1 μmol NADH per min by 1 mg of human ALDH2 protein. Molecular docking To visualize the interaction between the ALDH2 with activators Alda-1 and AD-5591 , the X-ray structure of human ALDH2 (PDB ID: 1NZX) and NAD + were used. Ligand energy was minimized using the PyRx 0.8 program before docking [55] . Three-dimensional models are generated by using the PyMOL v7.4 program [56] and the 2D protein-ligand interaction diagrams were generated by the LigPlot+ 2.2 program [57] . LC–MS/MS analysis of 4-HNE-modified proteins The protein samples were prepared with in-solution trypsin digestion. The peptides were desalted with C18 Zip Tip (Millipore, USA) and dry by vacuum centrifugation. The desalted and dried peptides were resuspended in 0.1% formic acid.LC-MS/MS analysis was performed on a NanoACQUITY UPLC system (Waters, USA) coupled to a high-resolution mass spectrometer (QE HF-X, Thermo Fisher Scientific). The peptides were injected into a trap column (Symmetry C18, 2 cm × 75 μm i.d.) and then separated in a 25 cm × 75 μm i.d. BEH130 C18 column (Waters, USA) on a gradient from 0% to 85% buffer B (buffer A, 0.1% FA H 2 O; buffer B, 0.1% formic acid in acetonitrile). The mass spectrometer was operated in data-dependent mode with the following acquisition cycle: an MS scan (m/z 350–1600) recorded at resolution R = 60,000 and MS/MS scans recorded at resolution R = 15,000, which were acquired by HCD (higher-energy C-trap dissociation fragmentation) with collision energy of 28.MS/MS spectra were searched with the Mascot engine (v2.6, Matrix Science) against the UniProtKB mouse protein database using the following parameters: a precursor peptide mass tolerance of 20 ppm and an MS/MS fragment tolerance of 0.02 Da with a maximum of two missed cleavage sites. The following modifications were made to the peptides: static carbamidomethylation on cysteine, variable oxidation on methionine, variable deamidation of asparagine or glutamine, and various 4-HNE modifications on cysteine, histidine and lysine. The cut-off threshold for acquiring significant peptide-to-spectrum matches was P < 0.05. The SI table of identified proteins is listed in Supplementary Table S2 and the all MASCOT mass spectrum analyses for identified 4-HNE adducted proteins by liquid chromatography tandem mass spectrometry (LC-MS/MS) were listed the Supplementary Data 1 . All raw mass spectrometry data to was uploaded to the MassIVE (Mass Spectrometry Interactive Virtual Environment) database ( https://massive.ucsd.edu/ProteoSAFe/static/massive.jsp ). The accession code is MassIVE00091724. Mitochondrial respiratory chain complex activity assay The mitochondrial complex spectrophotometric assays were carried out using published protocols [58] , [59] . Briefly, for mitochondrial complex activity assay and LC-MS/MS analysis, BAT was taken from 30-weeks Aldh2 WT or KI mice fed a HFHSD and homogenized in ice-cold mitochondrial isolation buffer (210 mM Mannitol, 70 mM sucrose, 1 mM EGTA, 0.5% BSA, 5 mM HEPES, pH7.2) by 10 strokes of the loose-fitting pestle of the Dounce homogenizer. The homogenate was spun at 800 × g and 4 °C for 10 min, and the supernatant was undergone another centrifugation at 8000 × g and 4 °C for 10 min. The pellet was re-suspended in STE buffer and measured protein concentration by Bradford assay. Complex I and complex II activities were measured spectrophotometrically by examining the decrease in absorbance due to the reduction of 2,6-dichlorophenolindophenol (DCPIP) at 600 nm. Activity was expressed in nanomoles of DCPIP reduction/min/mg protein (E = 19.1 mmol −1 ·cm −1 ). Complex III-specific activity and complex IV-specific activity were measured by monitoring the reduction of oxidized cytochrome C (IV) and oxidation of reduced cytochrome C (II) at 550 nm, respectively. The activity is expressed as a nanomole of reduced cytochrome of oxidized cytochrome C /min/mg protein (E = 18.5 mmol −1 ·cm −1 ). Immunoblots to detect 4-HNE-adducted proteins and Ucp1, Prdm16, Pgc1α, Dio2, and Cidea Samples prepared with Laemmli sample buffer and were separated by 10% SDS-PAGE gel and transferred to PVDF membrane. The membrane was blocked with 10% skim milk in PBST and incubated at 4 °C overnight with rabbit anti-4-HNE antibody (1:1000; cat. no. PAB1295, Abnova) and then with secondary antibodies with HRP(1:10000; cat. no. GTX26721, GeneTex). Immunoblots for Ucp1, Prdm16, Pgc1α, Dio2, Cidea, Hsp70, and Gapdh were performed using rabbit polyclonal anti-Ucp1 antibody (1:1000, cat. no. GTX10983, GeneTex), rabbit polyclonal anti-Prdm16 (1:1000, cat. no. ab106410, Abcam), rabbit polyclonal anti-Pgc1α antibody (1:1000, cat. no. NBP1-04676PCP, Novus), rabbit polyclonal anti-Dio2 antibody (1:1000, cat. no. GTX81072, GeneTex), rabbit polycloncal anti-Cidea (1:1000, cat. no. ab8402, Abcam), rabbit monoclonocal anti-Hsp70antibody (1:4000. cat. no.ab45133, Abcam), and rabbit polyclononal anti-Gapdh antibody (1: 5000,GTX100118, GeneTex). Oxygen consumption rate (OCR) Stromal vascular fraction was isolated from BAT of Aldh2 WT and KI mice at the age of 4–6 weeks and seeded to Seahorse XF24 v7 cell culture plates (Agilent) at approximate density of 20,000 cells per well and was then differentiated to primary brown adipocyte as described above. Briefly, on day7 of differentiation, cells were washed twice with Seahorse medium and maintained in Seahorse medium in CO 2 -less incubators. On the day before measurement, the medium was changed to DMEM medium containing 2% lipid-depleted FBS (cat. no. 26400044, Gibco), 3 mM glucose, and 2.5 mM glutamate. Basal OCR was determined by four measurements, followed by three measurements after each injection drug: oligomycin (2 μM), FCCP(carbonyl cyanide-p-trifluoromethoxyphenylhydrazone)(2 μM), Rotenone/Antimycin A (0.5 μM) using Seahorse XFe24 Analyzer (Agilent). OCR measurements of each stage were normalized to the cell number. Serum biochemistry Blood was collected from mice at the age of 24 weeks fasted for 4 h. Fasting serum adiponectin (cat. no. ab108785, Abcam), leptin (cat. no. DY498, R&D), free fatty acid (cat. no. LabAssay 294-63601, Wako), ethanol (cat. no. ab65343, Abcam), norepinephrine (cat. no. ab287789, Abcam), insulin (cat. no. 10-1247-01, Mercodia), and 4-HNE (cat. no. EEL-M2677, Elabscience) concentrations were measured using enzymatic or ELISA assay kits according to manufacturer’s instruction. Plasma triglycerides, and total cholesterol levels were measured using the FUJI DRI-CHEM clinical chemistry analyzer. Statistical analyses Two-tailed independent t -tests were used for comparing two independent groups. The Wilcoxon rank-sum test was used to compare data from RT-qPCR. Tests for linear trend were used for comparing difference among three genotypes. Data with multiple tests were analyzed with one-way analysis of variance (ANOVA) with Tukey’s post-hoc tests. Data with multiple time points were analyzed using repeated measures ANOVA. Energy expenditure among three genotypes was analyzed using the generalized linear model according to international guidance [60] , [61] . Energy expenditure (expressed as kcal/hr) was regressed on fat and lean mass using the command “glm” implemented in STATA 14.0 and the three genotypes were coded by allelic doses as 0,1, and 2 for WT, HE and KI mice, respectively [60] , [61] . All data are presented as mean and standard error (S.E.M.). The sample sizes of biological repeats were expressed as “n” and technical repeats were expressed as “in duplicates or triplicates”. The asterisks* indicates P < 0.05, ** indicates P < 0.01, *** indicates P < 0.001, and **** indicates P < 0.0001. Graphs were generated using GraphPad Prism 9.0. All two-sided P -values < 0.05 were considered statistically significant. Reporting summary Further information on research design is available in the Nature Portfolio Reporting Summary linked to this article.